Defective titanium dioxide single crystals exposed by high-energy {001} facets for efficient oxygen reduction The cathodic material plays an essential role in oxygen reduction reaction for energy conversion and storage systems. Titanium dioxide, as a semiconductor material, is usually not recognized as an efficient oxygen reduction electrocatalyst owning to its low conductivity and poor reactivity. Here we demonstrate that nano-structured titanium dioxide, self-doped by oxygen vacancies and selectively exposed with the high-energy {001} facets, exhibits a surprisingly competitive oxygen reduction activity, excellent durability and superior tolerance to methanol. Combining the electrochemical tests with density-functional calculations, we elucidate the defect-centred oxygen reduction reaction mechanism for the superiority of the reductive {001}-TiO 2− x nanocrystals. Our findings may provide an opportunity to develop a simple, efficient, cost-effective and promising catalyst for oxygen reduction reaction in energy conversion and storage technologies. Increasing energy demands have stimulated intense research on alternative energy conversion and storage systems with a high efficiency, low cost and environmental benignity. The oxygen reduction reaction (ORR) has a key role in metal-air batteries and polymer membrane electrolyte fuel cells [1] , [2] , but has become a bottleneck. ORRs traditionally require the exclusive use of platinum-based catalysts [3] , [4] . Owing to the high cost of Pt and declining activity, alternative catalysts based on non-precious metal oxides, for example, Fe 3 O 4 , Co 3 O 4 and so on, have been actively pursued [5] , [6] , [7] , [8] , [9] , [10] , [11] . TiO 2 is a widely used semiconductor because of its Earth abundance, low cost, no toxicity and high stability [12] . Thus, incorporating TiO 2 into energy conversion and storage systems is thus an attractive and promising idea. However, as a transition metal oxide, TiO 2 has not been considered as an efficient electrocatalyst because of its low conductivity and poor reactivity resulting from intrinsic insulating properties, for example, the wide bandgap energy ( E g =3.2 eV) (ref. 12 ). Up to now, several works have been reported on the use of TiO 2 for ORR, but an overall low activity is obtained [12] , [13] , [14] , [15] , [16] , [17] , [18] , [19] . Tremendous efforts have been made to improve TiO 2 electrochemical properties. The non-stoichiometric reduction of TiO 2 is known to substantially narrow the bandgap to the semiconductor level (usually below 2.0 eV) and thus increases the donor density and electric conductivities as well as the overall catalytic performance, because of the incorporated structural defects, that is, oxygen vacancy and Ti 3+ (refs 20 , 21 , 22 , 23 , 24 ). On the other hand, it is well documented that the ORR at MnO 2 proceeds through chemical oxidation of the surface Mn 3+ generated by the discharge of MnO 2 with O 2 splitting, and thus the catalytic activity is dependent highly on the electrochemical redox activity of these species [25] , [26] , [27] , [28] , [29] . Mn 3+ is the active valence state for ORR, owning to its single e g occupancy and thus the enhanced ability to stabilize ORR intermediates on the catalyst surface [30] , [31] , [32] , [33] . For other Mn-based oxides, the high ORR activities are also proposed to be a result of surface non-stoichiometry and the presence of surface Mn 3+ (ref. 29 ). In particular, Mn 3 O 4 with a unique mixed-valence state has been used as an active catalyst, since the coexistence of Mn 2+ , Mn 3+ and Mn 4+ facilitates the formation of defects, that is, vacancies, electrons and holes, which govern the electronic distribution of Mn 3 O 4 (refs 25 , 26 , 27 , 28 , 29 , 30 , 31 , 32 , 33 ). The surface atomic structure, physiochemical properties and catalytic activity of TiO 2 are also highly shape- and facet-dependent [34] . On the one hand, compared with randomly packed polycrystalline TiO 2 , the well-defined single crystals (SCs) with a high crystalline usually possess a much higher electronic conductivity and lower electron transfer resistance because of their continuous and ordered interior crystal structure, which favours the separation and transfer of reactive photocarriers as well as the overall catalytic performance [34] ; on the other hand, compared with the thermodynamically stable {101} facet of TiO 2 crystals with a low surface free energy (0.44 J m −2 ), the arrangement and category of constituent atoms on the high-energy {001} facet (0.90 J m −2 ) govern its unique geometrical and electronic structures, and its surface functional groups considerably affect its stability, adsorptive property and catalytic activity [34] . All these features make TiO 2 crystals with {001} facet highly efficient for various catalytic applications. Inspired by these informative results and the crystal similarity between TiO 2 and MnO 2 , we try to explore the feasibility of using the reduced non-stoichimetric TiO 2− x SCs containing the electro-conducting Ti 3+ species and oxygen vacancies as an ORR catalyst in energy conversion and storage systems. Herein, we first prepare the defective facet-controlled TiO 2− x SCs self-doped by oxygen vacancy via a facile solvothermal process, followed by a high-temperature thermal treatment in the reductive H 2 atmosphere; then systematically explore the TiO 2− x SCs as a catalyst for ORR by both electrochemical tests and density-functional calculations (DFTs); at last, the reasons for the observed superiority of TiO 2− x SCs in ORR are investigated. The facet- and defect-engineered TiO 2− x SCs exhibit a surprisingly high ORR activity, excellent durability and superior tolerance to methanol, owing to their defect-centred oxygen reduction mechanism. Morphological and structural properties of TiO 2− x SCs The morphology of the two prepared TiO 2 samples were highly truncated bipyramids of about 20 nm in diameter, with few one-dimensional nanorods randomly packed ( Fig. 1a,b and Supplementary Fig. 1 ). The lattice fringe spacing of 0.35 nm corresponded to the {101} planes, whereas the lattice fringe spacing of 0.47 nm corresponded to the {002} planes for the defective {001}-TiO 2− x SCs ( Fig. 1b ), indicating that the top/bottom surface exposed by truncation was bound by a {001} facet. Moreover, the angle labelled in the corresponding fast-Fourier transform image inset was 68.3°, which is in good agreement with the theoretical value of the angle between the {101} and {001} planes. The clear lattice fringes for the non-defective {001}-TiO 2 SCs with an interplanar lattice spacing of 0.35 and 0.47 nm corresponded to the (101) and (002) atomic planes, respectively ( Fig. 1d ), and the angle labelled in the fast-Fourier transform image was also 68.3°. These results suggest that the morphology, structure and facet exposing of the defective {001}-TiO 2− x SCs were well retained after high-temperature calcination under oxygen-rich atmosphere ( Fig. 1 ). 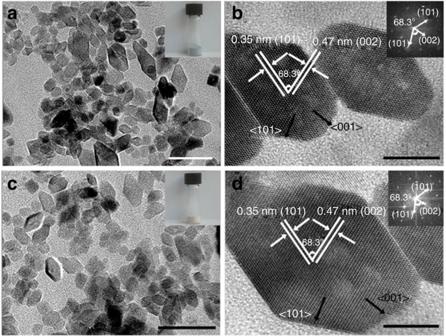Figure 1: Morphology and structure of different TiO2catalysts. Morphological (a,c) and structural (b,d) properties of the {001}-TiO2−xSCs and {001}-TiO2SCs, the insets ofbanddare their corresponding fast-Fourier transform patterns. Scale bars, 50 nm (a,c) and 10 nm (b,d). Figure 1: Morphology and structure of different TiO 2 catalysts. Morphological ( a , c ) and structural ( b , d ) properties of the {001}-TiO 2− x SCs and {001}-TiO 2 SCs, the insets of b and d are their corresponding fast-Fourier transform patterns. Scale bars, 50 nm ( a , c ) and 10 nm ( b , d ). Full size image In the given F-free nonhydrolytic alcoholysis route, {001}-TiO 2− x SCs were formed via the controlled and smooth hydrolysis of TiCl 4 in absolute ethanol [35] . Upon heating, ethanol was assumed to thermally react with dissolved oxygen and release water molecule (reaction 1), which coordinated to Ti 4+ cations to form titanium oxy/hydroxychloride complex from polymerization/condensation. Then, TiO 2 was formed with these complexes as intermediates (reaction 2). In this process, Cl − anions might act as the functional capping and shape controlling reagent to favourably reduce the surface energy difference between the {001} and {101} facets [34] . 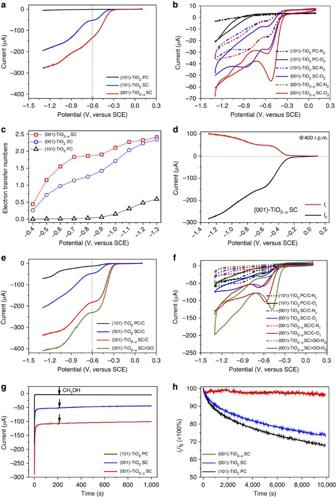Figure 2: ORR properties on different TiO2catalysts. Linear sweep voltammetry in O2-saturated 0.1 M aqueous KOH electrolyte solution at a scan rate of 10 mV s−1at 400 r.p.m. (a,e) and cyclic voltammetry in N2- and O2-saturated 0.1 M KOH at a scan rate of 10 mV s−1at 400 r.p.m. (b,f) electron transfer numbers calculated from the K-L model as a function of electrode potential (c) RRDE test on the defective TiO2−xin O2-saturated 0.1 M aqueous KOH electrolyte solution at a scan rate of 10 mV s−1at 400 r.p.m. (d) chronoamperometric responses obtained at −0.45 V in O2-saturated 0.1 M KOH at 200 r.p.m. with the addition of 10 vol.% methanol (g) and cathodic current stability obtained at −0.45 V in O2-saturated 0.1 M KOH at 200 r.p.m. (h). Supplementary Figure 2a shows the X-ray diffraction (XRD) patterns of the TiO 2 polycrystals (PCs), TiO 2 SCs and TiO 2− x SCs, in which the diffraction peaks highly matched those of anatase TiO 2 (JCPDS No. 21-1272), whereas the broadening of the diffraction peaks of the two facet-engineered samples could be attributed to their relatively smaller crystal size [34] . On the other hand, the reduced TiO 2− x sample displayed type IV nitrogen adsorption-desorption isotherms with hysteresis loops indicative of the mesoporous structure with narrow pore size distribution centred around 15.0 nm ( Supplementary Fig. 2b ). These mesopores were constructed by gathering nanoparticles into nanosheets, and the Brunauer–Emmett–Teller (BET) surface area was calculated as 47.0 m 2 g −1 from the nitrogen adsorption-desorption isotherms. Compared with the conventional F-mediated hydrothermal/solvothermal routes [34] , the prepared TiO 2 SCs possessed a smaller particle size and thus a higher surface area. These might provide more reactive sites for their catalytic applications, whereas the exposed percentage of high-energy {001} was relatively lower. Furthermore, the TiO 2− x SCs prepared using the Zn-mediated alcohothermal route in this work were very stable, and no obvious colour change was observed during its exposure in air even for over 1 year after their preparation. Their stability was comparable with the reduced TiO 2− x samples prepared by other methods [20] , [21] , [23] . The metallic Zn not only served as a functional reductant for the reductive formation of Ti 3+ , but also further stabilized the newly generated oxygen vacancies and hence Ti 3+ on the crystal surface and subsurface. It also increased the number of surface oxygen vacancies by weakening the surface-oxygen bonds and thus enhanced the overall catalytic activity of defective TiO 2− x polymorph [35] . ORR activity of TiO 2− x SC Figure 2 shows that the ORR curves on both the rotating disk electrode (RDE) and the rotating ring-disk electrode (RRDE) were in the order of {001}-TiO 2− x SCs > {001}-TiO 2 SCs > {101}-TiO 2 PCs. The onset potential on the {101}-TiO 2 PCs was beyond −1.0 V, whereas it positively shifted to approximately −0.4 V on the {001}-TiO 2 SCs and further to −0.3 V on the {001}-TiO 2− x SCs ( Fig. 2a ), when the crystals were self-doped by oxygen vacancies and Ti 3+ to form the reduced crystal structure. The cathodic current was also much higher on the facet- and defect-engineered TiO 2 sample ( Supplementary Table 1 ). At the given potential of −0.40 V (versus saturated calomel electrode (SCE)), the measured current density increased from 1.88 μA cm −2 on the {101}-TiO 2 PCs to 39.55 μA cm −2 on the {001}-TiO 2 SCs and further to 180.06 μA cm −2 on the {001}-TiO 2− x SCs ( Fig. 2a ). Figure 2: ORR properties on different TiO 2 catalysts. Linear sweep voltammetry in O 2 -saturated 0.1 M aqueous KOH electrolyte solution at a scan rate of 10 mV s −1 at 400 r.p.m. ( a , e ) and cyclic voltammetry in N 2 - and O 2 -saturated 0.1 M KOH at a scan rate of 10 mV s −1 at 400 r.p.m. ( b , f ) electron transfer numbers calculated from the K-L model as a function of electrode potential ( c ) RRDE test on the defective TiO 2− x in O 2 -saturated 0.1 M aqueous KOH electrolyte solution at a scan rate of 10 mV s −1 at 400 r.p.m. ( d ) chronoamperometric responses obtained at −0.45 V in O 2 -saturated 0.1 M KOH at 200 r.p.m. with the addition of 10 vol.% methanol ( g ) and cathodic current stability obtained at −0.45 V in O 2 -saturated 0.1 M KOH at 200 r.p.m. ( h ). Full size image The BET surface areas of the three involved TiO 2 samples exhibited no significant difference (47.0, 43.2 and 42.3 m 2 g −1 for {001}-TiO 2−x SCs, {001}-TiO 2 SCs and {101}-TiO 2− x PCs, respectively; Supplementary Figs 2–4 ), and their gathering modes were identical, implying that these TiO 2 samples have comparable electrochemical activities. Thus, the observed significant ORR superiority of the {001}-TiO 2− x SCs over the {001}-TiO 2 and {101}-TiO 2 polymorphs should be attributed mainly to the surface defect and {001} exposure ( Fig. 2 ), rather than other sources. Also, the identical chemical compositions, crystal morphologies and structures of the {001}-TiO 2− x SCs and {001}-TiO 2 SCs ( Fig. 1 and Supplementary Figs 2,4 and 5 ) rendered them comparable electrochemical ORR activities. This indicates that the observed ORR activity difference between the two TiO 2 samples dominantly originated from the defective crystal defects, oxygen vacancies and reduced Ti 3+ , rather than other sources. Moreover, the presence of coordination-unsaturated titanium sites increased the carrier density and facilitated the molecular diffusion of oxygen along the conducting crystal channels of the non-stoichiometric TiO 2− x SCs. The added Zn, served as both a reductant and a stabilizer, existed mainly in the form of ZnO clusters and dispersed on the TiO 2 surface owning to the larger ionic radii of Zn 2+ (0.88 Å) than Ti 4+ (0.745 Å) (ref. 35 ). However, the incorporation of such a small amount of foreign ZnO as impurity, that is, ∼ 0.80 atom % in this work ( Supplementary Fig. 5 ), would not bring about any ORR interference because of its low electrochemical activity as a wide bandgap n-type semiconductor [36] , [37] . The number of transferred electrons in ORR, n , was calculated from the slopes of straight lines at different potentials using the Koutecky–Levich model ( Supplementary Figs 6 and 7 ), and a continuous increase in n with the increasing overpotential was observed. Specifically, the calculated electron transfer number, n , was 0.44 at −0.4 V versus SCE and 2.41 at −1.3 V versus SCE for the defective {001}-TiO 2− x SCs ( Fig. 2c ), whereas only 0.26–2.34 and 0.00–0.59 for the perfect {001}-TiO 2 SCs and the commercial {101}-TiO 2 PCs, respectively. These calculation results indicate that the cathodic ORR on the three TiO 2 polymorphs under the given conditions, from −0.4 V to −1.3 V versus SCE, was dominantly via the two-electron pathway with a high overpotential. Such a two-electron pathway was further validated by the RRDE results ( Fig. 2d ) and is highly consistent with the DFT calculations. In the RRDE tests, the electrode modified with the defective {001}-TiO 2− x SCs generated a notable ring current, I r , over the whole potential range from the onset potential in 0.1 M KOH aqueous solution. This indicates the favourable and dominant generation of HO 2 − intermediate in the electrochemical reduction. Specifically, for the defective {001}-TiO 2− x SCs, the measured H 2 O 2 yield (HO 2 − % in alkaline solution) was 111.06% at the potential of −0.4 V versus SCE, and became 94.20% at −1.3 V versus SCE ( Supplementary Fig. 8 ). The calculated electron transfer number, n , from the RRDE tests varied in a range of 1.78–2.17 with the potential of −0.4 to −1.3 V versus SCE ( Supplementary Fig. 8 ). These RRDE results are consistent with the RDE results, suggesting that the ORR on the defective {001}-TiO 2− x SCs proceeded mainly via a two-electron pathway. Considering the low electric conductivity and poor dispersity of nano-sized metal oxide catalysts, some nano-structured carbonaceous supports are usually needed in ORR tests [18] . Herein, all the TiO 2 samples were mixed with the commercial Cabot carbon nanoparticles (Vulcan XC-72R, USA) as a conductive support. The same trend of ORR activity, {001}-TiO 2− x SCs/C>{001}-TiO 2 SCs/C > {101}-TiO 2 PCs/C, was also observed ( Supplementary Table 1 ). The {001}-TiO 2− x SCs was hydrothermally deposited on reduced graphene oxide (rGO) to form the {001}-TiO 2− x SCs/rGO hybrid, and it exhibited a further enhanced capacity for ORR ( Fig. 2e,f ). Interactions between rGO and metal oxide indicate a possible charge transfer across the interface depending on the hybrid interface spacing and the Fermi level difference, which might be the main reason for the enhanced ORR activity [10] , [11] . In addition, all linear sweep voltammetry (LSV) curves exhibited a slow current increase and no current plateau ( Supplementary Figs 6 and 9 ), indicating the two-electron reduction of O 2 to OOH − . All these results clearly indicate that both the exposed high-index {001} facet and the engineered oxygen vacancy contributed to the enhanced ORR activity of the TiO 2 catalyst. The long-time ORR stability was evaluated using chronoamperometric response at −0.45 V in O 2 -saturated 0.1 M KOH aqueous solution ( Fig. 2g,h ). The defective TiO 2− x SCs exhibited excellent stability, retaining more than 95% of the initial current even after 10,000 s, whereas both the TiO 2 SCs and TiO 2 PCs lost nearly 30% of the initial current. Moreover, all TiO 2 samples showed superior selectivity to ORR with no obvious current change after adding methanol. In addition, the TiO 2− x SCs also survived in the highly corrosive electrolyte (6 M KOH aqueous solution), demonstrating its high activity, favourable kinetics and excellent stability. The observed superior ORR stability of the defective TiO 2− x SCs should be attributed mainly to the excellent stability of the surface-engineered Ti 3+ species, because the metallic Zn not only served as a chemical reductant for the reductive formation of Ti 3+ but also further stabilized the newly generated oxygen vacancies and Ti 3+ on the crystal surface and subsurface [35] . The poor ORR catalytic stability of the TiO 2 PCs was probably owning to their anatase-rutile mixed crystal phase [38] , [39] . The above results clearly show that the ORR activity of TiO 2 was substantially enhanced by a simple facet- and defect-engineering strategy. It is noted that the prepared defect-engineered TiO 2− x with exposed high-energy {001} facets still exhibited a lower ORR activity than Fe 3 O 4 and Mn 3 O 4 (refs 10 , 32 ), the two most typical metal oxide ORR electrocatalysts, with a more negative onset potential of ca −0.30 V and a lower cathodic current density of ca 1.0 mA cm −2 ( Fig. 2a,b ). On the other hand, its ORR stability was much higher than the commercial Pt/C benchmark, as the chronoamperometric response remained intrinsically unchanged on the TiO 2− x while more than 20% decrease was observed on the Pt/C benchmark during the given 10,000 s (refs 4 , 5 , 9 ). Moreover, TiO 2 is intrinsically characterized of Earth abundance, low cost, high stability and environmental compatibility for industrial applications. Ti 3+ and its roles on TiO 2− x SCs The surface Ti oxidation state was probed by Fourier transform infrared (FTIR) spectroscopy, diffuse reflectance spectra, X-ray photoelectron spectroscopy (XPS), electron spin resonance (ESR) and Raman spectra, respectively ( Fig. 3 ). The FTIR spectrum exhibited two distinct -OH stretching bands at 3,400 and 1,632 cm −1 ( Fig. 3a ), indicating the presence of oxygen vacancies and/or reductive Ti 3+ as the reactive adsorption sites for water molecules and hydroxyl ions. The wider -OH absorption bands also suggest that the -OH groups experienced a more varied environment on the defective {001}-TiO 2− x SCs. In high-resolution XPS, an obvious shoulder appeared in the low-energy range (457.5–455.5 eV) of the Ti 2p spectrum, which might be attributed to Ti 3+ in the TiO 2 lattice ( Fig. 3c,d ) [22] . This was further confirmed by the ESR spectrum with the strong signals around g =1.95 and g =2.00, respectively [22] , but no significant signal indicative of surface Ti 3+ was observed at g =2.02 because of the surface oxidation ( Fig. 3e ). Moreover, the measured Raman spectra also confirmed the presence of more oxygen vacancies in the reduced TiO 2 SCs, owing to the positive peak shift, which was resulted from the modified geometric and surface structures ( Fig. 3f ) [23] . 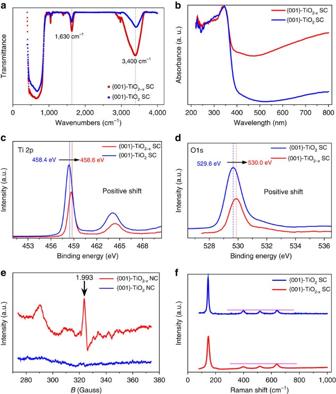Figure 3: Defects in TiO2−xSCs. Determination of defective Ti3+in the {001}-engineered TiO2−xSCs: FTIR (a), diffuse reflectance spectra (b), XPS (c,d), ESR (e) and Raman (f). Figure 3: Defects in TiO 2− x SCs. Determination of defective Ti 3+ in the {001}-engineered TiO 2− x SCs: FTIR ( a ), diffuse reflectance spectra ( b ), XPS ( c , d ), ESR ( e ) and Raman ( f ). Full size image In principle, the Ti 3+ species were generated from the reduction of Ti 4+ under reductive conditions and the in situ Ti 3+ -doped TiO 2 displayed oxygen vacancies because of the replacement of Ti 4+ by Ti 3+ in the lattice [20] , [21] , [22] , [23] , [24] . Meanwhile, the {001} facet contained more oxygen vacancies than the {101} facet, because each Ti in the {001} facet coordinated with 5 oxygen atoms, whereas each Ti in the {101} facet coordinated with either 5 or 6 oxygen atoms in the probability around 50% to 50% (ref. 34 ). The presence of Ti 3+ and the oxygen vacancies resulted in some new energy levels below the conduction band of the TiO 2 (refs 22 , 23 ), leading to an obvious spectral response in visible range ( Fig. 3b ). Such a photon excitation in the infrared region indicates that the formed Ti 3+ was dominantly derived from oxygen deficiency [24] . In addition, the oxygen-deficient TiO 2 SCs had different Raman spectra from the oxygen-free analogue, but they shared nearly the same XRD patterns. This result indicates that most oxygen deficiency-related Ti 3+ should mainly locate on the surface and subsurface of the crystals [21] . The presence of these structural defects played important roles in the electro-catalytic properties of the TiO 2− x . The enhanced visible light adsorption on the reduced TiO 2 SCs ( Fig. 3b ) indicates that the introduced new energy states by Ti 3+ self-doping mainly laid below the bottom of conductance band, and these electro-conducting Ti 3+ could significantly narrow the inherent bandgap and enhance the electrical conductivity ( Fig. 4a and Supplementary Fig. 10 ). In addition, both TiO 2 samples exhibited positive slopes as expected for n-type semiconductors, and a higher electron density was obtained for the TiO 2− x SCs from the slope of Mott–Schottky plot ( Fig. 4b ) [21] . Thus, although the TiO 2− x SCs were not the direct bandgap semiconductor ( Fig. 3b ), significant modifications of their electric structures occurred during the self-doping process, which contributes to their higher electron density. Moreover, all these enhanced electrochemical conductivity, reduced electron transfer resistance and improved interfacial capacity on the TiO 2− x SCs derived from the second semicircles in electrochemical impedance spectroscopy (associated with the fast reaction kinetics and considerable increases in the electrochemically accessible surface) are essential for an efficient ORR catalyst. 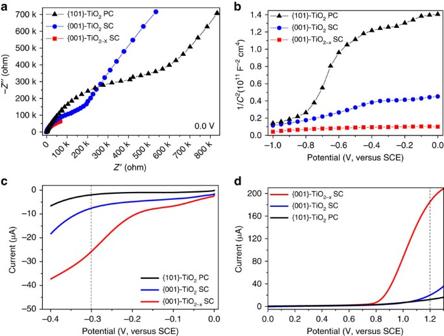Figure 4: Ti3+-induced properties of TiO2−xSCs. Role of defective Ti3+in the electronic and electrochemical properties of the {001}-engineered TiO2−xSCs: electrochemical impedance spectroscopy (a), Mott–Schottky (b), HER (c) and OER (d). Figure 4: Ti 3+ -induced properties of TiO 2− x SCs. Role of defective Ti 3+ in the electronic and electrochemical properties of the {001}-engineered TiO 2− x SCs: electrochemical impedance spectroscopy ( a ), Mott–Schottky ( b ), HER ( c ) and OER ( d ). Full size image Lowering the electrochemical overpotentials for both hydrogen evolution reaction (HER) and oxygen evolution reaction (OER) favours their efficient applications. In this work, both much reduced overpotentials and substantially enhanced currents were obtained on the defective {001}-TiO 2− x SCs for both HER and OER ( Fig. 4c,d ). For example, the cathodic current at the selected −0.3 V (versus SCE) and the anodic current at the selected +1.2 V (versus SCE) were −1.9 μA and 12.3 μA on the {101}-TiO 2 PCs, −7.5 μA and 20.2 μA on the {001}-TiO 2 SCs and −25.7 μA and 185.6 μA on the {001}-TiO 2− x SCs, respectively. The catalytic activity order of {001}-TiO 2− x SCs >{001}-TiO 2 SCs > {101}-TiO 2 PCs indicates that the introduction of defective oxygen vacancies uniformly into TiO 2 lattice and the exposed high-energy {001} facets could substantially improve their catalytic performance. Catalytic mechanism of TiO 2− x for ORR The ORR is affected by the chemical composition, elemental valence, crystal structure and surface state [5] , [6] , [7] , [8] , [9] , [10] , [11] . Also, the adsorption configuration of surface oxygen molecule and the corresponding strength of oxygen binding also impact with the ORR activities. In this work, the enhanced ORR activity on the defective {001}-TiO 2− x SCs might be highly associated with the single-crystalline structure, the exposed high-energy {001} facet and the Ti multiple valences caused by the defective oxygen vacancies ( Fig. 5 ). First, the significant enhancement of electric conductivity from both the continuous and ordered interior structure and the enhanced crystallinity should greatly favour fast electron transfer (that is, higher charge mobility) and reduce electrode polarization in ORR. Second, the exposed high-energy {001} facet with unique atomic, electronic and energetic structure could ensure its significant ORR activity because of its facet-mediated behaviours in dissociative adsorption and charge mobility [34] . Last, the active valence state of defective Ti 3+ originating from engineered oxygen vacancies could play a governing role in ORR and thus the enhanced ability to stabilize intermediates on catalyst surface owning to its single e g occupancy [40] . 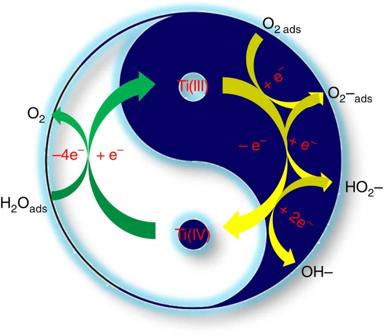Figure 5: Defect-centred ORR mechanism on TiO2−xSCs. The mixed-valence Ti species cycling between +3 and +4 states at oxygen vacancy sites in the defective TiO2−xSCs thermodynamically served as the reactive sites for cathodic oxygen reduction. Figure 5: Defect-centred ORR mechanism on TiO 2− x SCs. The mixed-valence Ti species cycling between +3 and +4 states at oxygen vacancy sites in the defective TiO 2− x SCs thermodynamically served as the reactive sites for cathodic oxygen reduction. Full size image In TiO 2 , the missed oxygen atom from the bulk or surface is taken by one or two ‘free’ electrons in the defective crystal, and the three nearest Ti atoms tend to relax away from the vacancy in order to strengthen their bonding with the rest of the lattice [20] . Thus, the defect-related properties mainly include structural, electronic, optical, dissociative adsorption and reductive properties [21] . For ORR, the chemical adsorption and dissociative activation of O 2 on the TiO 2 surface is a governing step, yet it has been well documented that both of the two processes are thermodynamically favoured only on the defective negative site, rather than the perfect neutral site [22] , [23] . In principle, the dissociated adsorption of O 2 on the defective oxygen vacancy could result in more efficient electron-transfer process and greater ORR kinetics because of the strong coupling between the adsorbate and the surface, and are intimately related to the overall catalytic performance. On the defective {001}-TiO 2− x SC, O 2 is first selectively adopted onto the defective subsurface oxygen vacancy with a much higher adsorption energy (reaction 3), as it only adsorbs onto the site where excess negative charge is available to form O-Ti bond; then, the chemically adsorbed O 2 could capture the free electrons located on oxygen vacancy site, simultaneously producing superoxide radical groups (reaction 4). The formation of these radical groups is effective to promote charge separation as well as the reduction of O 2 via either a two-electron pathway (reactions 5 and 6) or a 4-electron pathway (reactions 7 and 8), followed by the reduction of Ti 4+ to Ti 3+ (reaction 9). In this defect-centred ORR ( Fig. 5 ), the possible catalytic disproportionation of hydrogen peroxide occurs (reactions 7 and 8), which might be the overall rate-limiting step of the ORR. The DFT calculations further indicate that the four- and fivefold coordinated vacancy-surrounding titanium sites assume their respective role in oxygen adsorption and reactive activation, which lower the activation barrier and avoid catalytic poisoning. On the one hand, oxygen was found to be strongly bound onto the {001}-TiO 2− x with the highest adsorption energy of 2.28 eV ( Table 1 and Supplementary Note 1 ); on the other hand, based on the optimized geometry structures of adsorption configuration ( Fig. 6 ), the free energies ( G ) of key intermediates, O 2 − *, O 2 2– *, HOO − *, OH* and O* (*: adsorbed state; Supplementary Table 2 and Supplementary Note 1 ), and free energy changes (Δ G ) of each step of ORR, in Fig. 7a , were further calculated ( Supplementary Table 3 ) and the favourable energy profile is plotted on {001}-TiO 2− x ( Fig. 7b ). First, the Δ G of −3.297 eV for O 2 2– * formation is the lowest on {001}-TiO 2− x , compared with that of 3.945 and −2.478 eV on {101}-TiO 2 and {001}-TiO 2 ; second, for the overall rate-limiting ORR step of regenerating hydroxide from adsorbed oxide, {001}-TiO 2− x affords the lowest energy barrier of only 5.01 eV, compared with that of 10.58 and 7.55 eV on {101}-TiO 2 and {001}-TiO 2 ; at last, the total Δ G from adsorbed O 2 to 4OH − on {001}-TiO 2 , {001}-TiO 2− x and {101}-TiO 2 is −3.608 −7.741 and −2.806 eV, respectively. All these results not only confirm that {001}-TiO 2 was thermodynamically and kinetically more active than {101}-TiO 2 , but also show that oxygen vacancies on {001}-TiO 2− x effectively increased its catalytic activities. This conclusion is consistent with the electrochemical results ( Fig. 2 and Supplementary Figs 6 and 9 ). Table 1 Adsorption energy (Δ E ads ) for the three different adsorption configurations of O 2 on {001}-TiO 2 and {001}-TiO 2− x . 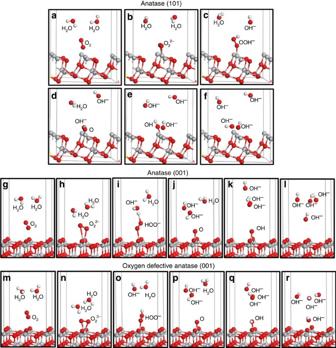Figure 6: Geometry structures of adsorption configuration. Optimized structures of each step in ORR on the {101}-TiO2, {001}-TiO2and {001}-TiO2−x. (a,g,m) Initial structure, (b,h,n) O22−*, (c,i,o) HOO−*, (d,j,p) O*, (e,k,q) OH* and (f,l,r) OH−, white, red and grey spheres indicate H, O and Ti atoms, respectively. Full size table Figure 6: Geometry structures of adsorption configuration. Optimized structures of each step in ORR on the {101}-TiO 2 , {001}-TiO 2 and {001}-TiO 2− x . ( a,g,m ) Initial structure, ( b,h,n ) O 2 2− *, ( c,i,o ) HOO − *, ( d,j,p ) O*, ( e,k,q ) OH* and ( f,l,r ) OH − , white, red and grey spheres indicate H, O and Ti atoms, respectively. 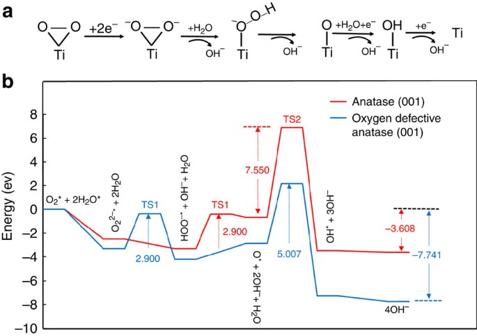Figure 7: ORR mechanism and energy profiles. DFT-calculated ORR mechanism on the anatase TiO2surface (a), and the energy profiles of ORR on the {001}-TiO2and {001}-TiO2−x, TS represents transition states (b). Full size image Figure 7: ORR mechanism and energy profiles. DFT-calculated ORR mechanism on the anatase TiO 2 surface ( a ), and the energy profiles of ORR on the {001}-TiO 2 and {001}-TiO 2− x , TS represents transition states ( b ). Full size image Although the further reduction of the generated peroxide on the defective {001}-TiO 2− x SCs showed a high-energy barrier of 5.01 eV, its Gibb’s free energy was −4.43 eV ( Supplementary Table 3 ), indicating that this step could spontaneously occur at room temperatures despite of a low reaction rate. Thus, the ORR reaction equilibrium was able to gradually shift to the reaction direction of deep oxygen reduction. Moreover, this theoretical ORR rate-controlling step with such a high-energy barrier for the subsequent reduction of the as-generated peroxide from the DFT calculations was further validated by both the RDE and RRDE tests. The calculated electron transfer number and peroxide percentage were ∼ 2.2% and ∼ 95%, respectively, even at a highly negative −1.3 V versus SCE on the defective {001}-TiO 2− x SCs ( Fig. 2c and Supplementary Fig. 8 ). Also, the geometric structural changes of this rate-controlling step were simple and lie in the last H 2 O dissociation and OH* generation. Thus, the series two-electron mechanism is the sole ORR pathway for this step. This mixed-valence in the defective TiO 2− x as the most active catalyst for defect-centred ORR is also consistent with the previous design principle for perovskite catalysts, especially on Mn-based oxides [25] , [26] , [27] , [28] , [29] , [30] , [31] , [32] , [33] . In addition, as the ORR involves the oxidation and reduction of surface-defective Ti species, the number and activity of these redox centres could be important factors to define the overall catalytic performance. In summary, we show that the new form of TiO 2 polymorph with defective crystal structure can be exploited as a promising ORR catalyst with a competitive activity, excellent durability and sufficient selectivity. The exposed high-energy {001} facets of the TiO 2 SCs is advantageous for oxygen interfacial adsorption and dissociative activation in ORR process. Moreover, the crystal oxygen vacancies and reductive Ti 3+ sites further guarantee a durable and facile ORR process via a defect-centred mechanism. Our findings might open up a new avenue for efficient energy conversion and storage technologies based on the Earth-abundant, scalable, non-precious metal catalysts. TiO 2− x SCs preparation The reduced TiO 2− x SCs engineered by the high-index {001} facet were prepared using a modified solvothermal method [34] . Briefly, at room temperature (10–15 °C), 2-ml TiCl 4 solution was slowly added into the absolute ethanol (40 ml) under vigorous stirring to form a transparent solution; then a given amount of metallic zinc powers with Ti/Zn molar ratio of 4:1 was added into the solution and magnetically stirred for over 1 h, in which process the solution colour gradually became blue; the obtained solution was immediately transferred into a 50-ml Teflon-lined stainless steel autoclave and was kept under 200 °C for 24 h; after this alcohothermal treatment and being cooled down to room temperature, the solution was subjected to high-speed centrifugation; the precipitate was collected and repeatedly washed with EtOH and water for several times, dried in vacuum at 60 °C and finally ground to obtain blue-coloured Ti 3+ self-doped TiO 2− x for use. For comparison, the commercial TiO 2 PCs with low-index {101} facet (P25, Degussa Co. , mean particle size of about 25 nm, anatase/rutile=80:20, BET surface area of 50 m 2 g −1 ) and the oxidized TiO 2− x SCs calcinated at 600 °C for 2 h under oxygen-rich atmosphere were used for reference. Material characterization The morphology and structure were characterized by high-resolution transmission electron microscopy (JEM-2100, JEOL Co.). XRD (X'Pert, PANalytical BV) was used to analyse the crystal structure. The diffuse reflectance spectra were measured on a ultraviolet–visible spectrophotometer (UV 2550, Shimadzu Co.). The chemical compositions were characterized using XPS (PHI 5600, Perkin-Elmer Inc.) and Raman spectrum (LABRAM-HR, JY Co.). The electronic state of Ti and O atoms were measured to provide structural information by ESR (JES-FA200, JEOL Co.). The surface area was measured using the BET method with a Builder 4200 instrument (Tristar II 3020M, Micromeritics Co.) at liquid nitrogen temperature. The infrared spectra were recorded between 4,000 and 400 cm −1 with a FTIR spectrometer (Magna-IR 750, Nicolet Instrument Co.) using a potassium bromide disc technique. Electrochemical characterization All electrochemical measurements were carried out in a home-made three-electrode system, with pure and modified TiO 2 SCs deposited on glass carbon as the working electrode, Pt wire as the counter electrode and Ag/AgCl (KCl, 3 M) as the reference electrode. Electrochemical impedance spectroscopy analysis was conducted by applying an AC voltage amplitude of 5 mV within the frequency range from 10 5 to 10 −2 Hz in 10 g l −1 NaCl aqueous solution; Mott–Schottky plots were measured in 0.1 M Na 2 SO 4 aqueous solution by impedance measurement at the fixed frequency of 1,000 Hz between the applied voltage range of 0–1 V; HER and OER were carried out in 0.5 M H 2 SO 4 aqueous solution and 0.1 M KOH aqueous solution, respectively, at a scan rate of 50 mV s −1 . ORR tests Electrochemical ORR, LSV and cyclic voltammetry measurements, on the glass carbon RDE (dimension of 5 mm, geometric surface area of 0.196 cm 2 ; Pine Research Instrumentation Inc.), were performed using a computer-controlled potentiostat (CHI 760D, CH Instrument) with a three-electrode glass electrochemical cell. The TiO 2 sample (2.0 mg) was dispersed in 2 ml absolute iso-propanol solvent. After applying ultrasonification for 30 min, 20 μl of the homogeneous suspension was dropped and the TiO 2 nanoparticles were adhered to the RDE using Nafion solution (5 μl, 0.05 wt. %) with a catalyst loading of ∼ 0.10 mg cm −1 . The ink was dried slowly in open air and the drying condition was adjusted by trial and error until a uniform catalyst distribution across the electrode surface was obtained [5] , [9] . The RDE loaded with different TiO 2 samples was used as the working electrode, an SCE as the reference electrode, and a Pt wire, as the counter electrode. The electrochemical ORR tests were conducted in either N 2 - or O 2 -saturated electrolyte (with 0.1 M KOH) at room temperature (10–15 °C). After purging O 2 or N 2 in the electrolyte for 30 min, the potential range was cathodically scanned between −1.3 and +0.1 V versus SCE at a scan rate of 10 mV s −1 . The LSV measurements were conducted at different rotating speeds from 400 to 1,600 r.p.m., using a Pine Model, whereas the cyclic voltammetry measurements were carried out without electrode rotating. In the ORR tests, the working electrode was cycled at least 15 times before electrochemical data were recorded, and a continuous flow of N 2 or O 2 was maintained to ensure saturation in supporting electrolyte. The ORR kinetic parameters are calculated using the Koutecky–Levich model: where i is the measured current, i k is the kinetic current and ω is the electrode rotation rate. The theoretical value of the Levich slope ( B ) is evaluated from the following equation: where n is the electron transfer number in ORR, F is the Faradic constant (96,485 C mol −1 ), C O2 is the saturated oxygen concentration in 0.1 M KOH aqueous solution (1.2 × 10 −6 mol cm −3 ), D O2 is the oxygen diffusion coefficient (1.73 × 10 −5 cm 2 s −1 ) and ν is the kinematic viscosity of the solution (0.01 cm 2 s −1 ). Electrochemical ORR measurements on the glass carbon RRDE (disk electrode: dimension of 5 mm, geometric surface area of 0.196 cm 2 ; Pine Research Instrumentation Inc.) were carried out by the same procedures as on the RDE. The disk electrode was scanned cathodically at a rate of 10 mV s −1 and the ring potential was kept constant at +0.3 V versus SCE. The HO 2 − percentage and the electron transfer number, n , are determined by the following equations: where I d is disk current, I r is ring current and N is current collection efficiency of the Pt ring, which was determined to be 0.40 from the reduction of K 3 Fe[CN] 6 . DFT calculations DFT calculations were carried out using the ultrasoft pseudopotential for electronic–ion interactions and generalized gradient approximation with the Predew–Burke–Ernzerhof exchange for exchange-correlation functional in the supercell approach as implemented in CASTEP program [41] , [42] . The convergence criteria was set out to be express , and the tolerances of the energy was 1 × 10 −3 eV per cell. The norm-conserving pseudopotential was constructed using the pseudopotential generator implemented in CASTEP. The energy cutoff of 750 eV for the plane wave basis was used throughout the study. The Brillouin zone integration was obtained with variable numbers of k -points, depending on the unit cell size and shape, generated by the Monkhorst-pack algorithm. Phonon dispersion and density of states were computed using the method of Finite displacement. The linear synchronous transit/quadratic synchronous transit methods were employed to search for the transition state structure and acquire the activation energy ( E a ) of ORR [43] . The adsorption energy (Δ E ads ) was calculated to estimate the strength of a molecule–surface interaction and to seize the most energetically stable adsorption model. The Δ E ads could be expressed as: where the total energy values E system , E surf , E react are relative to supercells simulating a molecule interacting with anatase TiO 2 surfaces, the surfaces and an isolated molecule in the vacuum, respectively. The Gibb’s free energy difference (Δ G ) of each elementary reaction was given by the following equation: where Δ E is the total energy change, directly obtained from DFT calculations, ΔZPVE is the change in zero-point energies, T is temperature (298.15 K) and Δ S is the change in entropy. For the surface models, a vacuum region of 15 Å was embedded along surface to avoid the unwanted interaction between the slab and its period images. The {001}-TiO 2 surface had fivefold coordinated Ti atoms only, interconnected at the surface by two-coordinate bridging oxygen atoms, whereas the {101}-TiO 2 surface exhibited a sawtooth-like corrugation consisting of 5-coordinate and 6-coordinate Ti atoms as well as 2-coordinate and 3-coordinate oxygen atoms. In addition, according to the experiments, the {001}-TiO 2− x surface was constructed from the perfect {001}-TiO 2 surface model with a subsurface oxygen vacancy. How to cite this article: Pei, D.-N. et al . Defective titanium dioxide single crystals exposed by high-energy {001} facets for efficient oxygen reduction. Nat. Commun. 6:8696 doi: 10.1038/ncomms9696 (2015).